Trehalose glycopolymer resists allow direct writing of protein patterns by electron-beam lithography Direct-write patterning of multiple proteins on surfaces is of tremendous interest for a myriad of applications. Precise arrangement of different proteins at increasingly smaller dimensions is a fundamental challenge to apply the materials in tissue engineering, diagnostics, proteomics and biosensors. Herein, we present a new resist that protects proteins during electron-beam exposure and its application in direct-write patterning of multiple proteins. Polymers with pendant trehalose units are shown to effectively crosslink to surfaces as negative resists, while at the same time providing stabilization to proteins during the vacuum and electron-beam irradiation steps. In this manner, arbitrary patterns of several different classes of proteins such as enzymes, growth factors and immunoglobulins are realized. Utilizing the high-precision alignment capability of electron-beam lithography, surfaces with complex patterns of multiple proteins are successfully generated at the micrometre and nanometre scale without requiring cleanroom conditions. Direct-write patterning of biomolecules at micrometre and nanometre length scales has the potential to enable pattern generation with fewer fabrication steps. In addition, direct-write approaches facilitate the generation of geometrically complex multicomponent patterns at the micrometre and nanometre scale with the advantage compared with indirect strategies that there is no limit in the number of different proteins that can be patterned. Yet despite these advantages, only a few examples have been reported to directly pattern biomolecules on surfaces at the submicron scale [1] , [2] , [3] , [4] , [5] . The majority has employed physical deployment onto surfaces using an atomic force microscopy (AFM) tip such as dip-pen lithography or polymer-pen lithography; these techniques involve pressing or flowing the material onto a surface and do not require a resist. This is because the approaches in which radiation is utilized, such as electron-beam lithography (EBL) require the development of resists that are not only water soluble, but also protect the biomolecules from denaturation during irradiation and other processing steps. These requirements have significantly hindered the investigation of direct-write biomolecule patterns by techniques such as EBL. EBL is a maskless patterning technique that generates user-designed complex patterns at high resolution. Although a serial technique, EBL offers nanometre-scale alignment capability, which enables interfeature spacings that are so small that different protein features may be touching or arrayed one on top of the other allowing for complex, multiplexed patterns [6] . The majority of protein patterning by EBL has been accomplished by indirect approaches [6] , [7] , [8] , [9] , [10] , [11] , because the high-vacuum and high-energy radiation inactivates proteins. Indeed, the harsh conditions required have been exploited to pattern by selective ablation of proteins on electron-beam exposure [7] , [8] . Thus far, there have only been two resists that have been employed for direct protein pattering by EBL; proteins bacteriorhodopsin and green fluorescent protein were patterned using poly(acrylic acid) and silk as resists [1] , [3] . In both the studies, the authors noted that the proteins used had exceptionally stable structures, which enabled them to be stable under harsh conditions of EBL. Herein, we describe a resist material, a trehalose glycopolymer that stabilizes a variety of proteins including antibodies and sensitive growth factors to repeated exposure to vacuum and to electron beams allowing for direct write by EBL, as well as multiplexing. The latter is critical for full realization of the technology in applications such as sensors. Trehalose glycopolymer patterning by EBL The trehalose glycopolymer explored for EBL has a polystyrene backbone and trehalose side chains (polystyrenyl ether trehalose or poly(SET), Fig. 1 ). This particular backbone was chosen because polystyrene is known as a negative-tone EBL resist [11] , [12] . Thus, it was anticipated that the polymer would crosslink under electron-beam irradiation. Indeed, on exposure to electron beams, this polymer was crosslinked and covalently bound to the silicon/silicon dioxide surfaces. Overexposure was observed at doses above 70 μC cm −2 , while the patterns looked sharp at an area dose of 40 μC cm −2 ( Supplementary Fig. 1 ). These doses are much lower than that required for patterning polystyrene enabling much faster patterning which makes poly(SET) a cost-effective resist. The polymer likely crosslinks to the surface and to other polymer chains by a radical crosslinking mechanism similar to that observed for other polymers such as poly(ethylene glycol) (PEG) [6] , [9] . 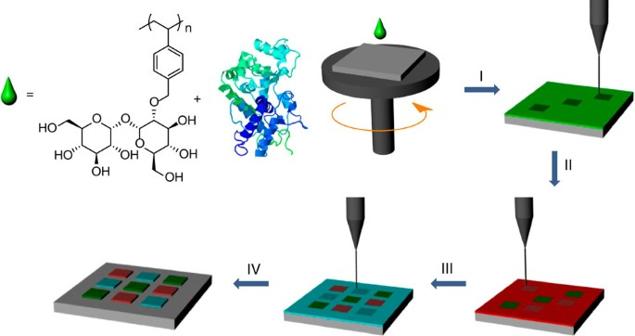Figure 1: EBL process for multiple protein patterns. I, spin coating with poly(SET)-protein-1 solution and writing of the first layer. II, rinsing of the unexposed poly(SET)-protein-1 followed by spin coating poly(SET)-protein-2, alignment to the first layer and writing of the second layer. III–IV, multiple protein patterns are obtained by repeated spin coating, alignment, writing and rinsing steps. All of the steps including EBL were performed outside the cleanroom. Protein structure from PDB# 1W4Y. Figure 1: EBL process for multiple protein patterns. I, spin coating with poly(SET)-protein-1 solution and writing of the first layer. II, rinsing of the unexposed poly(SET)-protein-1 followed by spin coating poly(SET)-protein-2, alignment to the first layer and writing of the second layer. III–IV, multiple protein patterns are obtained by repeated spin coating, alignment, writing and rinsing steps. All of the steps including EBL were performed outside the cleanroom. Protein structure from PDB# 1W4Y. Full size image The trehalose side chains impart significant aqueous solubility to the polymer; the polymer solubility in water is greater than 815 mg ml −1 . Trehalose is accumulated in large amounts by many plants and animals under desiccation stress and dramatically increases the resistance of these organisms, as well as cells and biomolecules to such environmental stresses [13] , [14] , [15] . We recently reported that polymers with trehalose side chains provide superior protection to proteins against heating and freeze drying in solution than does trehalose [16] , [17] . The polymers combine the advantageous properties of the osmolyte and non-ionic surfactant class of stabilizers into one material. Because it was not clear if poly(SET) could stabilize proteins in the solid form and against harsh electron-beam irradiation exposure and vacuum steps, our next experiments were to determine if the polymer could stabilize proteins to the EBL conditions. Direct-write protein patterning with poly(SET) The process for generating protein patterns is outlined in the top of Fig. 1 . An aqueous solution containing the protein to be patterned and poly(SET) is first spin-coated onto silicon substrates. Then, the poly(SET)-protein patterns are generated by EBL. Horseradish peroxidase (HRP) was used as a model protein to investigate the effect of protein concentration, polymer concentration on the obtained patterns, and also to determine the optimal area dose (energy) required to obtain the HRP-poly(SET) patterns ( Fig. 2a , Supplementary Figs 1 and 2 ). The signal-to-noise ratio (S/N) for each condition was determined using the images of patterns stained with a fluorescent anti-HRP antibody. When the protein concentration was varied at a constant poly(SET) concentration, the immunostained patterns showed very high fluorescence signal (S/N>150) for concentrations at or above 10 μM. The observed increase in S/N values could be related to higher protein concentration in the resulting gel, which also would increase the stability of the protein [18] . The polymer concentrations were then investigated. By studying the S/N values, it was determined that the optimal polymer concentration was 0.5 wt %. At lower concentration (0.3 wt %), a weak antibody signal was observed either because the polymer concentration was not high enough to protect the protein or because the starting film thicknesses were smaller (see Supplementary Table 1 for film thicknesses). On the basis of these results, 0.5 wt % polymer concentration and 10 μM final protein concentration were chosen for further experiments. Importantly, the data indicate that during crosslinking of poly(SET), the protein was immobilized in the newly formed features, likely either by physical entrapment within the network or by covalent binding to the network. The data also suggest that the antibody binding site of HRP was not significantly influenced by the EBL process. 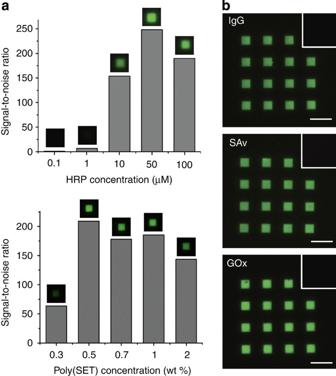Figure 2: Proteins patterned by direct electron beam using poly(SET) as a resist. (a) Effect of HRP and poly(SET) concentration on S/N ratio of poly(SET)-HRP patterns. Top: Poly(SET) concentration was set to 0.5 wt% and bottom: HRP concentration was 10 μM; in each case S/N calculated for optimal dose is shown. (b) Fluorescence micrographs of fluorescent antibody-stained poly(SET)-IgG, poly(SET)-SAv, poly(SET)-GOx. Insets show that fluorescent antibodies do not bind nonspecifically to poly(SET) patterns that did not contain respective proteins. Scale bars, 25 μm. Figure 2: Proteins patterned by direct electron beam using poly(SET) as a resist. ( a ) Effect of HRP and poly(SET) concentration on S/N ratio of poly(SET)-HRP patterns. Top: Poly(SET) concentration was set to 0.5 wt% and bottom: HRP concentration was 10 μM; in each case S/N calculated for optimal dose is shown. ( b ) Fluorescence micrographs of fluorescent antibody-stained poly(SET)-IgG, poly(SET)-SAv, poly(SET)-GOx. Insets show that fluorescent antibodies do not bind nonspecifically to poly(SET) patterns that did not contain respective proteins. Scale bars, 25 μm. Full size image To determine the ability of poly(SET) to stabilize a range of proteins and for later multiprotein patterning, we chose glucose oxidase (GOx), immunoglobulin G (IgG) and streptavidin (SAv), in addition to HRP, because these proteins are utilized in a wide range of bionanotechnological applications such as diagnostic assays and biosensors, and also are readily available. First, dose tests for the different proteins were performed ( Supplementary Fig. 6 , first column). The highest S/N was obtained at an area dose of 45 μC cm −2 for HRP, GOx and SAv, while for IgG the optimal dose was 25 μC cm −2 . After staining the protein-poly(SET) patterns that had been written at their optimal writing doses, high fluorescent signals (S/N>120 for all the proteins used) were observed ( Fig. 2b ). To rule out nonspecific binding of antibodies to poly(SET), we incubated poly(SET) patterns (written without protein) with all the fluorescently labelled antibodies that have been used in this work. In all of the cases, no pattern was visible by fluorescence microscopy ( Fig. 2b insets). Therefore, the fluorescence signals seen in Fig. 2b are due to specific antigen–antibody interactions. Importantly, successful staining of IgG shows that their recognition property is preserved. Therefore, direct writing of IgGs with trehalose glycopolymers is a promising method of generating antibody arrays for diagnostics and proteomics studies. Moreover, when four successive HRP patternings were applied on the same substrate, the fluorescence intensity of the first layer was comparable to the fourth layer (exposed to four EBL cycles, Fig. 3a ). This suggests that exposure of the formed poly(SET)-protein patterns to repeated vacuum-vent and rinsing cycles did not have an adverse effect on the protein structure, a requirement for multicomponent patterning by EBL. The poly(SET)-HRP patterns generated by EBL were also visualized by scanning electron microscopy. 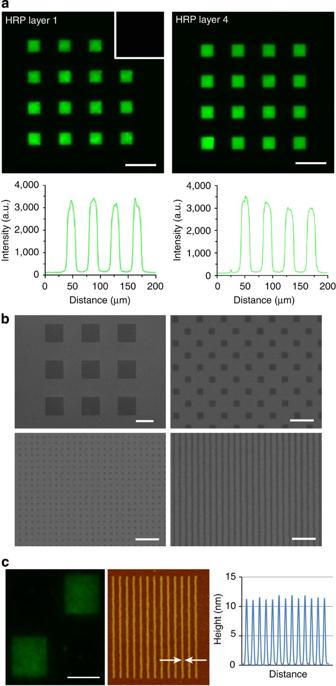Figure 3: Multiple layers and nanopatterning. (a) Poly(SET)-HRP patterns (first and fourth layer written on the same substrate are shown) and fluorescence intensity profiles drawn along second row of squares from the top. Inset shows that fluorescent antibodies do not bind nonspecifically to poly(SET) patterns that did not contain respective proteins. Scale bars, 25 μm. (b) Scanning electron microscopy micrographs showing micro- and nanopatterns of poly(SET)-HRP. Scale bars are 10 μm (top left), 2 μm (top right) and 1 μm (bottom left and bottom right). (c) HRP patterns with nanometre line spacing showing fluorescence, AFM and height profile. Scale bar, 5 μm and arrows indicate line width of 110 nm. Figure 3b shows square patterns with 10-μm and 500-nm side lengths as well as sub-100 nm dots and lines of poly(SET)-HRP. Nanosized protein features were also observed by AFM as shown in Fig. 3c (magnified AFM shown in Supplementary Fig. 3 ). HRP was patterned with 110-nm line widths with 200 nm spacing before fluorescent antibody binding. Because the nanometre features were arrayed close together, the overall fluorescence was observable ( Fig. 3c left) demonstrating that the HRP in the nanometre features still bound antibody. Figure 3: Multiple layers and nanopatterning. ( a ) Poly(SET)-HRP patterns (first and fourth layer written on the same substrate are shown) and fluorescence intensity profiles drawn along second row of squares from the top. Inset shows that fluorescent antibodies do not bind nonspecifically to poly(SET) patterns that did not contain respective proteins. Scale bars, 25 μm. ( b ) Scanning electron microscopy micrographs showing micro- and nanopatterns of poly(SET)-HRP. Scale bars are 10 μm (top left), 2 μm (top right) and 1 μm (bottom left and bottom right). ( c ) HRP patterns with nanometre line spacing showing fluorescence, AFM and height profile. Scale bar, 5 μm and arrows indicate line width of 110 nm. Full size image Activity of the patterned proteins Observing the protein activity is a critical component to prove direct-write capabilities and for protein arrays. The IgG exhibited activity; it still bound to antibodies as described above. The activity of SAv patterns was assessed by a biotin-binding assay ( Supplementary Fig. 4a ). After generating poly(SET)-SAv patterns, the substrates were incubated with an eight-arm PEG–biotin. Subsequent incubation with AF488-labelled SAv was used to detect the surface-bound PEG–biotin in a sandwich assay format. The poly(SET)-SAv patterns showed strong fluorescence signal after incubation with PEG–biotin and fluorescent SAv indicating that the written SAv molecules retained their biotin-binding properties and thus the biological activity. No signal was observed when only poly(SET) was patterned or when the PEG–biotin incubation step was skipped. These control experiments confirmed that the observed fluorescence signal for poly(SET)-SAv patterns was indeed due to the specific interaction of SAv with biotin. The activity of poly(SET)-HRP patterns was assessed using a tetramethylbenzidine assay. The observed activity of poly(SET)-HRP patterned substrates was higher (0.037±0.009 a.u., P <0.035) than that measured for control substrates that had been spin-coated with poly(SET)-HRP and charged into scanning electron microscopy chamber but not exposed to electron beams and washed (0.019±0.005 a.u.). The signal observed for control substrates is likely due to nonspecifically adsorbed protein that was not removed during the washing step. Importantly, poly(SET) was not a substrate for tetramethylbenzidine and did not influence the measurements. Finally, the activity of poly(SET)-GOx patterns were visualized by the formation of gold nanoparticles on the generated patterns as a result of reduction of gold ions by glucose oxidase ( Supplementary Fig. 4b ) [19] . The data together demonstrate that the direct write of these proteins with poly(SET) resulted in bioactive protein patterns. Patterning relevant proteins that are components in the extracellular matrix (ECM) are valuable for preparing bioactive surfaces in cell–material interaction applications and for understanding fundamental cell–ECM interactions. For example, Spatz and coworkers [20] have shown that nanometre interfeature spacings of integrin-binding peptides are critical to cell adhesion. Thus, important ECM proteins, such as fibronectin, and signalling molecules such as basic fibroblast growth factor (bFGF) and vascular endothelial growth factor (VEGF) were patterned with poly(SET) ( Supplementary Fig. 5 ). Particularly, bFGF is known for its remarkable instability [21] , [22] . The ability to both stabilize as well as pattern and present bioactive signalling molecules as shown here has great potential. Stabilization effectiveness of poly(SET) Several compounds including amino acids [23] , sugars [24] and polymers [25] have been shown to improve protein stability. Therefore, the effectiveness of PEG and trehalose to stabilize HRP, IgG, GOx and SAv were compared to poly(SET). First, the optimal writing dose (the dose that gave the highest S/N) was determined for each excipient protein ( Supplementary Fig. 6 ), then the S/N values were determined for each excipient-protein pattern that had been written at the optimal dose ( Fig. 4 and Supplementary Fig. 7 ). In all cases, significantly higher fluorescence signals were observed for protein patterns that had been written with poly(SET) compared with those that had been written with PEG, trehalose or with no additive ( Fig. 4a and Supplementary Fig. 7 ). 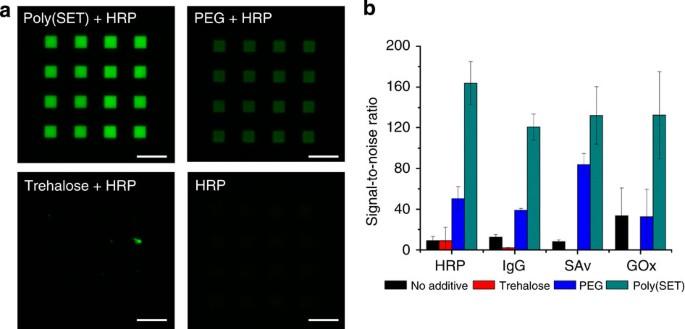Figure 4: Effect of different excipients on protein patterning. (a) Fluorescence micrographs of HRP patterned with poly(SET), PEG, trehalose or without additive after staining with AlexaFluor 488 goat anti-HRP. Scale bars, 25 μm. (b) S/N ratios calculated for different proteins patterned with different excipients. S/N values were significantly higher for poly(SET) patterns compared with other excipients (P<5.3 × 10−5, <6.6 × 10−5, <0.019, <0.038 for HRP, IgG, SAv, GOx, respectively). Figure 4b shows that the S/N values for poly(SET) (average S/N=120–164 for different proteins) were consistently higher than PEG (average S/N=32–84 for different proteins). Since both polymers can be crosslinked by an electron-beam irradiation, the lower signals observed for PEG are due to a less efficient stabilization capability or to a less efficient grafting efficiency of this polymer compared to poly(SET). It has been observed that trehalose glycopolymers are superior stabilizers to PEG when exposed to other stresses (heat and lyophilization) in solution [16] , [17] . In the case of trehalose and no additive, the fluorescence signals were very low; this is to be expected since the ablation of proteins by electron beams is known, and furthermore trehalose does not crosslink during the electron-beam process. Figure 4: Effect of different excipients on protein patterning. ( a ) Fluorescence micrographs of HRP patterned with poly(SET), PEG, trehalose or without additive after staining with AlexaFluor 488 goat anti-HRP. Scale bars, 25 μm. ( b ) S/N ratios calculated for different proteins patterned with different excipients. S/N values were significantly higher for poly(SET) patterns compared with other excipients ( P <5.3 × 10 −5 , <6.6 × 10 −5 , <0.019, <0.038 for HRP, IgG, SAv, GOx, respectively). Full size image To rule out any differences in the amount of protein coated onto the surface of the substrates during spin coating with different excipients, we prepared substrates by placing a 5-μl drop of protein-excipient solution onto the chips and letting it spread over the surface instead of spin coating (film thicknesses provided as Supplementary Table 2 ). After drying these substrates under vacuum, the patterns were generated by EBL and stained with fluorescent antibodies ( Supplementary Fig. 8 ). When the solution was spread onto the substrates and dried, higher S/N values (average S/N ranged from 70 to 184, Supplementary Fig. 9 ) were obtained with PEG compared with those obtained for the spin-coated substrates (average S/N ranged from 32 to 51). Nevertheless, the average S/N for poly(SET) was the highest in all cases (average S/N ranged from 197 to 240). It should be noted that trehalose itself does not form patterns on the surface up to high dosages (1,000 μC cm −2 ) and adding trehalose to PEG gave results similar to PEG alone. Thus, covalent attachment of the trehalose to the polystyrene resist is critical to observe the stabilization of proteins. In an effort to understand the mechanisms of protein stabilization by poly(SET) during EBL process, we investigated the effect of radicals formed on electron-beam irradiation and the effect of high-vacuum conditions ( Supplementary Fig. 10 ). When poly(SET)-HRP-coated substrates having different concentrations of ascorbic acid (Vitamin C) as a radical scavenger were exposed to electron beams, an increase in the fluorescence intensity was observed with increasing ascorbic acid concentrations ( Supplementary Fig. 10a ). The calculated S/N values increased from 69±10 to 192±12 when the ascorbic acid concentration was increased from 0 to 1 mM. This suggests that likely the ascorbic acid molecules reduce the amount of inter- and intramolecular crosslinking reactions by scavenging the formed radicals and help in preservation of protein structure. As expected, the minimum dose required for crosslinking also increased with an increasing concentration of ascorbic acid and eventually a concentration of 10 mM prevented crosslinking and thus pattern formation. The S/N value for no ascorbic acid was lower than shown in Fig. 2 because to prevent overexposure of the ascorbic acid samples, the samples without additive were underexposed. We also investigated the activity of HRP with different excipients after being exposed to high-vacuum conditions for 4 h. HRP loses activity just on exposure to the vacuum, but in the presence of trehalose, PEG or poly(SET) the activity of HRP is much higher ( Supplementary Fig. 10 ). PEG and poly(SET) were equally as good at stabilizing the protein to vacuum. Thus, the results observed when patterning by EBL must be a result of poly(SET)s superior ability to stabilize against exposure to electron-beam irradiation. Interestingly, in the presence of both poly(SET) and ascorbic acid, the highest activity for HRP was observed, indicating that ascorbic acid helps stabilization of HRP during desiccation. Multiple protein micro- and nanopatterns Patterning of multiple biomolecules at micrometre and nanometre length scales is important for a myriad of applications. For example, miniaturized biomolecule arrays are valuable in the development of rapid and highly sensitive diagnostic assays, biosensors and in the discovery of novel drugs, biomarkers or drug targets. In addition, they are powerful tools in studying, elucidating and modulating the cell behaviour on bioactive surfaces that are crucial for tissue engineering and regenerative medicine [26] , [27] , [28] . Most of these applications require multiple proteins to be immobilized at high resolution and in close proximity with precision, a unique capability of EBL. While utilization of orthogonal chemistries or highly specific supramolecular interactions enables indirect patterning of more than one protein on the same surface by EBL, the ultimate number of different biomolecules that can be immobilized is limited by the number of orthogonal reactions available. In addition, these approaches require efforts to functionalize the proteins with complementary functional groups. Therefore, direct-write patterning of proteins is desirable to generate complex patterns of multiple proteins. To demonstrate the applicability of the direct EBL technique in generating multiplexed antibody arrays in close proximity, contiguous micropatterns of multiple proteins were generated using human, chicken and mouse immunoglobulins ( Fig. 5 ). First, poly(SET)-human IgG patterns were written to create a checkerboard patterns or arrays of crosses. After removing the non-crosslinked polymer and protein from the surface by washing and spin coating with the poly(SET)-chicken IgG, a complementary pattern was written. Then, a third layer was written with mouse IgG. Sequential staining of the patterns with respective labelled antibodies allowed visualization of tricolour checkerboard or cross-array patterns. It can be seen that fluorescent antibodies are mainly confined to the areas where respective IgGs had been written without significant cross-reactivity. 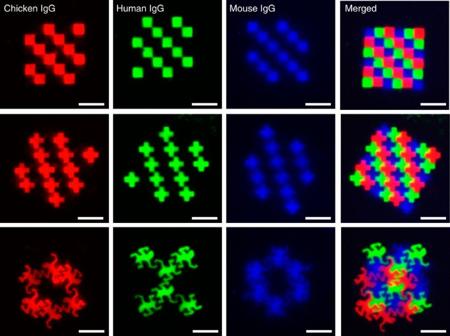Figure 5: Multiple protein micropatterns. Fluorescence micrographs showing fluorescent antibody-stained individual IgG patterns written with poly(SET): chicken IgG (red channel), human IgG (green channel) and mouse IgG (blue channel). The merged images show all the patterned IgGs forming a tricolour checkerboard, a cross-array and a design inspired by M.C. Escher’s work ‘Reptiles’. Scale bars, 25 μm. Figure 5: Multiple protein micropatterns. Fluorescence micrographs showing fluorescent antibody-stained individual IgG patterns written with poly(SET): chicken IgG (red channel), human IgG (green channel) and mouse IgG (blue channel). The merged images show all the patterned IgGs forming a tricolour checkerboard, a cross-array and a design inspired by M.C. Escher’s work ‘Reptiles’. Scale bars, 25 μm. Full size image With EBL, it is possible to make patterns based on user-created designs (so called arbitrary patterns). To illustrate that complex multicomponent patterns can be obtained with the direct protein patterning technique, a patterned inspired by M.C. Escher’s work ‘Reptiles’ was generated with the three IgGs in the same manner as described above. The resulting patterns demonstrate the complexity of patterns possible, as well as the ability to pattern different proteins in close proximity. Different shapes with nanometre-sized features were also generated with the three different IgGs ( Fig. 6a,b ). The resulting images showcase the nanoscale resolution patterning and alignment capabilities of this technique. 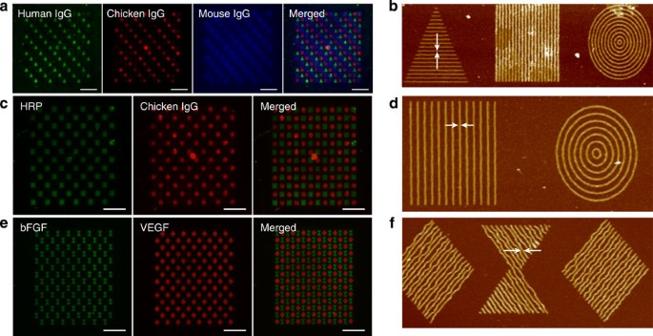Figure 6: Multiple protein nanopatterns. (a) Fluorescent micrographs showing fluorescent antibody-stained individual IgG patterns with human IgG (triangles, green channel), chicken IgG (circles, red channel) and mouse IgG (squares, blue channel) and merged. (b) AFM of corresponding patterns with arrows indicating line width of 80 nm. (c) Fluorescent micrographs of antibody-stained HRP (squares, green channel) and chicken IgG (circles, red channel) and merged image. (d) AFM of corresponding HRP and chicken IgG stained patterns with arrows indicating line width of 110 nm. (e) Fluorescent micrographs of antibody-stained bFGF (hourglass shapes, green channel) and VEGF (diamonds, red channel) and merged imaged. (f) AFM of corresponding VEGF and bFGF patterns with arrows indicating line width of 100 nm. Scale bars, 25 μm. Figure 6: Multiple protein nanopatterns. ( a ) Fluorescent micrographs showing fluorescent antibody-stained individual IgG patterns with human IgG (triangles, green channel), chicken IgG (circles, red channel) and mouse IgG (squares, blue channel) and merged. ( b ) AFM of corresponding patterns with arrows indicating line width of 80 nm. ( c ) Fluorescent micrographs of antibody-stained HRP (squares, green channel) and chicken IgG (circles, red channel) and merged image. ( d ) AFM of corresponding HRP and chicken IgG stained patterns with arrows indicating line width of 110 nm. ( e ) Fluorescent micrographs of antibody-stained bFGF (hourglass shapes, green channel) and VEGF (diamonds, red channel) and merged imaged. ( f ) AFM of corresponding VEGF and bFGF patterns with arrows indicating line width of 100 nm. Scale bars, 25 μm. Full size image Multicomponent nanopatterning is also important for generating high-density, high-sensitivity arrays that could be very useful in fields such as proteomics, diagnostics and biosensors. Such patterns could also be used to generate complex surfaces to investigate cell behaviour and to control cell shape for instance surfaces that present multiple integrin-binding proteins and growth factors to direct stem cell lineage or surfaces that present a gradient of a bioactive molecule [26] , [27] , [28] , [29] , [30] , [31] , [32] . To investigate this capability, multiprotein nanoarrays of HRP with chicken IgG ( Fig. 6c,d ) and VEGF with bFGF ( Fig. 6e,f ) were written. Each feature was composed of ~100 nm wide lines and the overall pattern in these arrays covered a dimension of 5 × 5 μm 2 . For HRP and chicken IgG, the individual elements comprising the protein pattern shape had a centre-to-centre distance of 400 nm, while the HRP and IgG shapes were separated by a distance of 3 μm for better visualization of the individual elements in the arrays. For VEGF and bFGF, the centre-to-centre distance of the individual elements was set to 250 nm, while each VEGF and bFGF pattern was separated by a distance of 500 nm. The data show that indeed nanoarrays are possible. Such patterns could be very useful in generating bioactive surfaces for investigating fundamental questions about protein–protein interactions, as well as studying the effect of geometry on cell behaviour or the effect of multivalency in cell behaviour. In conclusion, the use of a polystyrene backbone trehalose glycopolymer has been shown to allow the direct patterning of bioactive proteins by providing stabilization to high-energy radiation and vacuum conditions during EBL. The versatility of this direct patterning approach has been demonstrated by generating complex, multicomponent micro- and nanopatterns of proteins. Although protein patterns were demonstrated, it is readily envisioned that this approach can be extended to other biomolecules such as DNA, carbohydrates and so on. Thus, we expect that this biomolecule patterning technique will find broad application in different disciplines and will be important in designing bioanalytical assays, biosensors, microreactors and bioactive interfaces for cell culture. Materials Silicon wafers were obtained from Cemat Silicon S.A., Poland. Trehalose was purchased from The Healthy Essential Management Corporation (Houston, TX). Sheep anti-glucose oxidase antibody was obtained from Abcam. Human, chicken and mouse IgGs and the fluorescent antibodies AF488 goat anti-HRP, AF488 donkey anti-human IgG, AF594 donkey anti-chicken IgG were purchased from Jackson ImmunoResearch. AF350 donkey anti-mouse IgG, AF488 donkey anti-rabbit IgG, AF488 goat anti-sheep IgG were bought from Invitrogen. 2- O -(4-vinylbenzylidene)-α,α-trehalose and poly(SET) were prepared by following our literature procedure [17] . All the other chemicals were obtained from Sigma-Aldrich and Fisher Scientific unless otherwise stated. For generating multicomponent patterns, silicon chips with gold alignment marks were fabricated by standard photolithography, metal evaporation and lift-off techniques [6] . Effect of polymer and protein concentration Silicon substrates were cleaned with freshly prepared piranha solution (3:1 H 2 SO 4 /H 2 O 2 , Caution! Piranha solution reacts violently with organic materials). After washing with 10 × 200 ml of MilliQ water and drying under a stream of air, the cleaned substrates were spin-coated (500 r.p.m., 5 s; 1,000 r.p.m., 5 s; 2,000 r.p.m., 20 s; or 4,000 r.p.m. for 10 s) with a 30-μl solution containing poly(SET) and HRP. To investigate the effect of protein concentration, 25 μl of poly(SET) (0.5 wt % in H 2 O) was mixed with 5 μl of protein solution (ranging from 0.60 to 600 μM in D-PBS) leading to final protein concentrations ranging from 0.1 to 100 μM. Poly(SET)-HRP patterns were generated using a JC Nabity e-beam lithographic system (Nanometre Pattern Generation System, version 9.0) modified from a JEOL JSM-6610 scanning electron microscope. The pattern files for EBL were designed using DesignCAD Express 16 software. An accelerating voltage of 30 kV was used, with a beam current of ~15 pA, a spot size of 30–40 nm. Square patterns (10 μm) were written at a dose range from 5 to 80 μC cm −2 . After electron-beam exposure, any non-crosslinked polymer on the chips was washed away with D-PBS containing 1 mM of Tween 20 (PBS-Tween); the surfaces were then stained with AF488 goat anti-HRP antibody (10 μg ml −1 in PBS-Tween). To investigate the effect of polymer concentration, 25 μl of poly(SET) (0.3–2 wt % in H 2 O) was mixed with 5 μl of protein solution (60 μM in D-PBS) leading to a final protein concentration of 10 μM. Patterns were written at doses ranging from 3 to 96 μC cm −2 and stained as described above. Single-protein patterning with different excipients A dose test was performed for each protein-excipient pair (HRP, GOx, sheep IgG or SAv with poly(SET), PEG, M n =14,000 g mol −1 , trehalose or no additive) to determine the optimal area dose; the dose that resulted in highest S/N ratio after antibody staining. The spin-coating solutions contained 25 μl of poly(SET) (0.5 wt % in H 2 O) or molar equivalents of PEG or trehalose (molar equivalent to trehalose in poly(SET)) and 5 μl of protein (60 μM in D-PBS) leading to a final protein concentration of 10 μM. On each substrate, a 4 × 4 array of 100 μm 2 squares were written four times at doses ranging from 5 to 80 μC cm −2 ( n =3). After antibody staining was performed as described above, S/N ratios were calculated for each dose and the optimal area dose was determined for each protein excipient. Once the optimal dose was determined for each protein excipient, a total of 64 squares measuring 100 μm 2 squares were written on each substrate at the predetermined optimal dose ( n =3) and then stained with respective antibodies (10 μg ml −1 in PBS-Tween). To compare the different excipients, S/N ratios were calculated for 3 × 64 squares that had been written for each protein excipient. Patterning of multiple proteins and immunostaining Silicon substrates with gold alignment marks were piranha cleaned and spin-coated with a 30 μl solution of poly(SET) (25 μl, 0.5 wt % in H 2 O) and protein (5 μl of protein 30 μM in D-PBS) as described above. After the first pattern had been written with human IgG, the substrates were washed with PBS-Tween followed by a very brief rinsing with MilliQ H 2 O. After alignment to the first layer, a complementary pattern was written with chicken IgG. The third layer was written with mouse IgG. The generated patterns were visualized by immunofluorescence staining. The substrates were sequentially incubated with fluorescently labelled donkey anti-human, donkey anti-chicken and donkey anti-mouse IgGs (30 min, 10 μg ml −1 in PBS-Tween). In between the incubation steps, the substrates were washed with PBS-Tween solution. HRP and chicken IgG multi-patterned substrates were prepared similarly as described above. In brief, the alignment substrates were spin-coated with a solution containing 25 μl of 0.5 wt% poly(SET) in H 2 O and 5 μl of 60 μM HRP or IgG in D-PBS. The first layer patterned was HRP followed by chicken IgG with PBS-Tween washes in between the patterning and spin-coating steps. For visualization by immunofluorescence, the patterns were sequentially stained with Alexa Fluor 488 anti-HRP and Alexa Fluor 594 anti-chicken IgGs (30 min, 10 μg ml −1 in PBS-Tween) with PBS-Tween washes in between the incubation steps. VEGF and bFGF multi-patterned substrates were prepared similarly by first spin coating and patterning VEGF followed by bFGF. The spin-coating solutions contained 25 μl of 0.5 wt% poly(SET) in H 2 O and 5 μl of a 2-mg ml −1 VEGF or bFGF solution in D-PBS. After patterning, the substrates were sequentially incubated with biotinylated anti-bFGF, mouse anti-VEGF, SAv-conjugated Alexa Fluor 488 and Alexa Fluor 594 anti-mouse IgG (30 min, 10 μg ml −1 in PBS-Tween) and washed with PBS-Tween in between incubation steps. Fluorescence microscopy The immunostained patterns were visualized by fluorescence microscopy using a Zeiss Axiovert 200 fluorescent microscope equipped with an AxioCam MRm monochrome camera, and pictures were acquired and processed using AxioVision LE 4.6 software. NIH ImageJ software was used to calculate the S/N ratio as (signal—background)/s.d. of background. Atomic force microscopy Height characterization of patterns was imaged on a Bruker Dimension Icon AFM using Peak Force tapping mode with ScanAsyst Air probes. AFM imaging was performed on a scan size of 25.0 μm, with a scan rate of 0.7 Hz and 512 samples per line. Film thickness measurements Film thicknesses from spin-coating solutions of 5 μl HRP (60 μM in PBS) and 25 μl poly(SET) (0.3, 0.5 or 1 wt%) were measured. In addition, 0.5 wt% of poly(SET) and 0.1–100 μM HRP were evaluated. Separately, the drop-coated thickness of HRP with different additives was evaluated. Ellipsometry was performed using a Gaertner LSE ellipsometer equipped with a 633 nm HeNe laser fixed at a 70° incidence angle. The silicon oxide on the piranha-cleaned silicon wafer was measured and fitted using the refractive index of Palik ( n 1=0.54264, k 1=0.00) and silicon as substrate ( n 1=3.589, k 1=0.016). The measurement was repeated on the same wafer after spin coating the HRP and poly(SET) solution. The subsequent protein and polymer layer was fitted using values for the previously obtained silicon oxide thickness and an additional Cauchy layer model ( n 1=1.45, k 1=0.01). A minimum of 15 measurements were performed at three different locations and the values were then averaged. How to cite this article: Bat, E. et al . Trehalose glycopolymer resists allow direct writing of protein patterns by electron-beam lithography. Nat. Commun . 6:6654 doi: 10.1038/ncomms7654 (2015).